Skp2 suppresses apoptosis inRb1-deficient tumours by limiting E2F1 activity One mechanism of tumour suppression by pRb is repressing E2F1. Hence, E2f1 deletion diminishes tumorigenesis following Rb1 loss. However, E2F1 promotes both proliferation and apoptosis. It therefore remains unclear how de-repressed E2F1 promotes tumorigenesis. Another mechanism of pRb function is repressing Skp2 to elevate p27 to arrest proliferation. However, Skp2 deletion induced apoptosis, not proliferation arrest, in Rb1 -deficient pituitary tumorigenesis. Here we show that Rb1 deletion induces higher expression of E2F1 target genes in the absence of Skp2. E2F1 binds less cyclin A but more target promoters when Rb1 is deleted with Skp2 knockout or p27T187A knockin, suggesting that stabilized p27 prevents cyclin A from binding and inhibiting E2F1. In Rb1 -deficient pituitary tumorigenesis, Skp2 deletion or p27T187A mutation converts E2F1’s role from proliferative to apoptotic. These findings delineate a pRb-Skp2-p27-cyclin A-E2F1 pathway that determines whether E2F1 is proliferative or apoptotic in Rb1 -deficient tumorigenesis. Classic RB1 deficiency-induced tumorigenesis follows the two-hit paradigm. Typical patients inherit a null allele of RB1 (and therefore is RB1 +/− ), develop retinoblastoma with full penetrance and the tumour cells are invariably RB1 −/− . This paradigm is modelled in melanotrophs in pituitary intermediate lobe (IL) of Rb1 +/− mice. A major approach to studying pRb employs in vitro experiments to identify pRb targets and Rb1 +/− mice to determine the physiological roles of the targets in Rb1 -deficient tumorigenesis [1] , [2] . The E2F transcription factors are the best-studied pRb targets. pRb binds and represses E2F to inhibit expression of E2F target genes, many of which encode for proteins that promote proliferation. Knockout (KO) of E2f1 , E2f3 or E2f4 partially inhibits pituitary tumorigenesis in Rb1 +/− mice [3] , [4] , [5] . Thus, E2F1, E2F3 or E2F4 each plays demonstrable roles in promoting Rb1 -deficient tumorigenesis. These experiments have added value for E2F1 since it can also induce apoptosis. Experiments with Rb1 +/− mice demonstrate that deregulated E2F1 plays a proliferative role. Skp2, first identified as a cyclin A-binding protein in transformed cells (S phase kinase binding protein 2) [6] and later established as the substrate recruiting subunit of SCF Skp2 E3 ubiquitin ligase [7] , [8] , is another pRb target. pRb represses Skp2 messenger RNA expression [9] , [10] , promotes Skp2 protein degradation [11] and prevents Skp2 from recruiting phosphorylated p27 (p27T187p) for ubiquitination [12] . When re-expressed in pRb-deficient tumour cells in culture, pRb represses Skp2 to elevate p27 protein levels to arrest cell cycle in G1/S with a faster kinetics than its repression of E2F (ref. 12 ). When combined with Skp2 KO, pituitary tumorigenesis in Rb1 +/− mice was prevented [13] . To study how Skp2 deletion prevented tumorigenesis, we used POMC-Cre to delete Rb1 in the entire pituitary IL [13] . We expected that Rb1 deletion in the absence of deregulated Skp2 would elevate p27 to inhibit melanotroph proliferation and, therefore, prevent tumorigenesis. Surprisingly, we found increased apoptosis, such that by 7 weeks of age the entire pituitary IL was ablated. This phenotype explained the prevention of pituitary tumorigenesis in Rb1 +/− mice but raised questions about how this was achieved. Since E2F1 possesses both proliferative and apoptotic activities, it has been proposed that E2F1 must be restrained once the cells have progressed into S phase to prevent its apoptotic activity from manifesting [14] . One means of restraining E2F1 in S phase was suggested by the ability of cyclin A, which is expressed to higher levels from mid-late S phase, to inhibit E2F1 activity by binding to it [15] , [16] , [17] , [18] . Other means include degradation of E2F1 protein by SCF Skp2 , SCF Slmb and CRL4 Cdt2 (refs 19 , 20 , 21 ). Here we describe a pRb-Skp2-p27-cyclin A-E2F1 pro-survival mechanism to limit E2F1 activity for Rb1 -deficient pituitary tumorigenesis. Skp2 and Rb1 co-deletion further upregulates E2F targets To study how Skp2 and Rb1 co-deletion induced apoptosis in pituitary melanotrophs, we determined whether mouse embryonic fibroblasts (MEFs) of the same genotypes could serve as a model. We used Adeno-Cre to delete Rb1 in Rb1 lox/lox MEFs. Deletion of Rb1 by Adeno-Cre was confirmed by genotyping ( Supplementary Fig. 1a ). Controls included Adeno-GFP infection of Rb1 lox/lox MEFs and Adeno-Cre infection of Rb1 +/+ MEFs. Same as pituitary studies, Skp2 deletion was by germline KO. For brevity, we will use Skp2;Rb1 DKO MEFs to indicate Adeno-Cre-infected Skp2 −/− ;Rb1 lox/lox MEFs, and use Skp2 KO MEFs to indicate Adeno-GFP-infected Skp2 −/− ;Rb1 lox/lox MEFs and so on. We used DNA content fluorescence-activated cell sorting to measure apoptosis (sub-G1 cells, Fig. 1a ). Consistent with previous findings [22] , Skp2 KO induced more cells with 4N DNA content (G2/M) and 8N DNA content (fully duplicated chromosomes failed to divide into daughter cells) compared with wild-type (WT) MEFs. Skp2 KO MEFs also contained several folds more sub-G1 cells than WT MEFs, but apoptosis remained below 1% of the population. Deletion of Rb1 did not change cell cycle or apoptosis profiles as previously reported [23] , but increased apoptosis population by 20-fold in Skp2;Rb1 DKO MEFs. We confirmed this effect by staining with anti-cleaved caspase-3 and TdT-mediated dUTP nick-end labelling (TUNEL; Supplementary Fig. 1b–e ). We conclude that MEFs are susceptible to Skp2 and Rb1 co-deletion-induced apoptosis, but the extent of apoptosis might be smaller than what was observed in pituitary melanotrophs [13] . 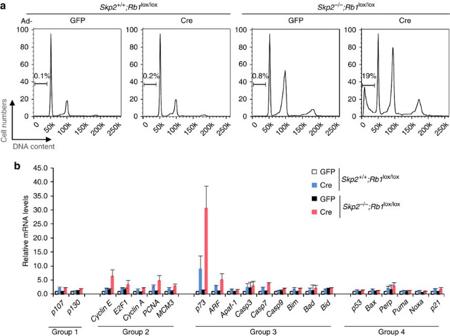Figure 1: Co-deletion ofSkp2andRb1induces apoptosis and higher expressions of E2F target genes than deletion ofRb1in MEF. (a) Following propidium iodide staining, indicated MEFs were analysed by fluorescence-activated cell sorting. Sub-G1 cell population sizes are marked. (b) RT–qPCR (three replicates) was performed with the same set of MEFs to measure mRNA expression of four groups of genes. Relative mRNA abundance is shown with abundance in WT MEFs set to 1.0. Data are expressed as average (mean)±s.e.m. Figure 1: Co-deletion of Skp2 and Rb1 induces apoptosis and higher expressions of E2F target genes than deletion of Rb1 in MEF. ( a ) Following propidium iodide staining, indicated MEFs were analysed by fluorescence-activated cell sorting. Sub-G1 cell population sizes are marked. ( b ) RT–qPCR (three replicates) was performed with the same set of MEFs to measure mRNA expression of four groups of genes. Relative mRNA abundance is shown with abundance in WT MEFs set to 1.0. Data are expressed as average (mean)±s.e.m. Full size image We next used reverse transcription quantitative PCR(RT–qPCR) to measure the expression of E2F target genes in two pairs of MEFs: WT versus Rb1 KO, and Skp2 KO versus Skp2;Rb1 DKO ( Fig. 1b ). The test genes were divided into four groups. Group 1 contains p107 , an E2F target gene and is upregulated in germline Rb1 −/− MEFs. Following Cre-mediated Rb1 deletion, this compensation was not immediately significant [23] . The other Rb family member p130 is not an E2F target gene [24] and is included in this group for comparison. Group 2 includes typical E2F target genes that promote proliferation. Group 3 is for E2F target genes with apoptotic activity. Arf is included in this group, since it links E2F activation to p53-dependent apoptosis [25] . p53-activated apoptotic genes constitute group 4, which also includes a canonical p53 target gene p21 for comparison. Expression values were normalized with that of glyceraldehyde 3-phosphate dehydrogenase (GAPDH) in the same samples. Expression in WT MEFs was then set to 1.0 as the reference point and other three genotypes were presented relative to it. The results reveal that Skp2 KO slightly changed expression of the tested genes around the reference point (white and black columns). Rb1 deletion in Rb1 KO MEFs induced two- to threefold increases in many E2F target genes. Interestingly, expression of p73 increased fourfold more than the rest ( Supplementary Fig. 2a shows an enlarged view of the blue columns with horizontal axis crossing at 1.0). In this framework, expression of most of these genes showed further increases when Rb1 was deleted in Skp2;Rb1 DKO MEFs (red columns). 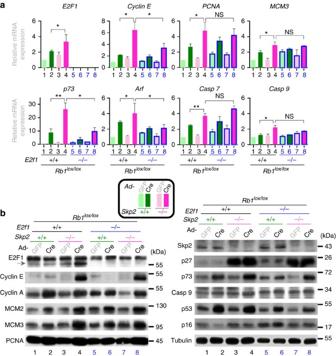Figure 2: Increased and further increased expressions of certain E2F target genes wereE2f1dependent. (a) RT–qPCR results for the indicated genes in various MEFs. Colours were used to help convey patterns of sample arrangement. As shown by the decoder in the middle of the figure, green indicatesSkp2+/+and pink indicatedSkp2−/−; lighter colours are for GFP expression and darker colours for Cre expression. Blue frames are added to the columns to indicate combinedE2f1KO. Experiments were performed more than three times. Data are expressed as average (mean)±s.e.m. Unpairedt-tests were performed, NS,P>0.05, *P<0.05, **P<0.01. (b) Western blots of same sets of MEFs as ina. Uncropped scans are shown inSupplementary Fig. 10. Supplementary Figure 2b shows the fold increases in Skp2;Rb1 DKO cells over the fold increases in Rb1 KO cells. Expressions of many genes in group 2 and group 3 showed further increases. Since p73 expression was already increased about ninefold by Rb1 deletion, Skp2 co-deletion further increased it to 30-fold higher over the reference point. Thus, Skp2 co-deletion with Rb1 further enhances the expression of many E2F target genes, and these included both proliferative and apoptotic genes. Skp2 and Rb1 co-deletion leads to higher E2F1 activity Among the genes whose expression was further increased by Skp2 and Rb1 co-deletion, p73 is likely an E2F1 target gene [26] , [27] , and E2F1 can induce apoptosis in diverse scenarios [28] , [29] . E2F2 and E2F3 can also induce or contribute to induce apoptosis [30] , [31] , [32] . To determine the role of E2F1 in the further increased expression of the E2F target genes, we generated Rb1;E2f1 DKO MEFs and found that expression of cyclin E, PCNA, MCM3, caspase 7 and caspase 9 increased similarly to those found in Rb1 KO MEFs ( Fig. 2a , green columns 1, 2 with 5, 6), indicating that other E2F family members were (also) de-repressed following Rb1 deletion to increase expression of these E2F target genes. In comparison, the expression of p73 and Arf was increased less in Rb1;E2f1 DKO MEFs than in Rb1 KO MEFs, revealing that E2F1 played a more important role in their increased expression following Rb1 deletion. More importantly, the further increases in their expression in Skp2;Rb1 DKO MEFs were not observed in Skp2;Rb1;E2F1 TKO MEFs ( Fig. 2a , pink columns 3, 4 and 7, 8). Furthermore, although increase in cyclin E expression by Rb1 deletion was not E2f1 dependent (green columns), its further increase by Skp2 and Rb1 co-deletion was (pink columns). These findings suggest that E2F1 was further activated by Skp2 co-deletion to further increase the expression of cyclin E, p73 and Arf. Figure 2: Increased and further increased expressions of certain E2F target genes were E2f1 dependent. ( a ) RT–qPCR results for the indicated genes in various MEFs. Colours were used to help convey patterns of sample arrangement. As shown by the decoder in the middle of the figure, green indicates Skp2 +/+ and pink indicated Skp2 −/− ; lighter colours are for GFP expression and darker colours for Cre expression. Blue frames are added to the columns to indicate combined E2f1 KO. Experiments were performed more than three times. Data are expressed as average (mean)±s.e.m. Unpaired t -tests were performed, NS, P >0.05, * P <0.05, ** P <0.01. ( b ) Western blots of same sets of MEFs as in a . Uncropped scans are shown in Supplementary Fig. 10 . Full size image We next determined whether gene expression changes at mRNA levels translated to protein levels. We noticed that E2F1 protein was not increased by Rb1 deletion ( Fig. 2b , lanes 1 and 2), suggesting that E2F1 could be under negative regulation by protein degradation [19] , [20] , [21] . We found that E2F1 protein levels were very slightly increased in Skp2 KO MEFs compared with WT MEFs (lanes 1 and 3), but significantly increased in Skp2;Rb1 DKO MEFs compared with Skp2 KO MEFs (lanes 3 and 4), indicating that E2F1 mRNA increase is the primary mechanism for further increase in E2F1 protein. Further increases in protein levels of cyclin E, MCM3 and p73 were also consistent with the further increases in their mRNA levels by Skp2 and Rb1 co-deletion. Compared with mRNA levels, the dramatic further increases in cyclin E protein levels (lane 4) might suggest that protein stabilization also played a role [22] , [33] , while the less dramatic increases in p73 protein levels compared with its mRNA levels might suggest post-transcriptional negative regulation of p73 (refs 34 , 35 ). E2f1 KO mostly prevented further increases in p73 protein and partially prevented further increases in cyclin E protein in Skp2;Rb1;E2f1 TKO MEFs. Increases in cyclin A protein were not affected by E2f1 deletion, indicating that other E2F family members (also) play important roles, similar to the regulation of MCM3. For p53 protein, its dramatically more increase in protein levels than in its mRNA levels ( Fig. 1b ) by Rb1 deletion may represent the activation of the typical pRb-E2F1-Arf-MDM2-p53 safeguard [36] . We determined whether findings from MEFs were applicable to pituitary IL. We harvested pituitaries from 2.5-week-old mice. At this age, pituitary IL of the Skp2 −/− ;POMC-Cre,Rb1 lox/lox genotype was of similar sizes as WT IL. We performed immunofluorescence staining for E2F1, MCM3, cyclin A and p73, and found increased staining for these proteins following Rb1 deletion in IL, further increases of them following Skp2 co-deletion, and lack of increases when E2f1 was additionally deleted ( Fig. 3 ). Staining for p73 was further tested by immunohistochemistry ( Supplementary Fig. 3 ). Thus, co-deletion of Skp2 enhanced E2F1 activation in pituitary IL over deletion of Rb1 . 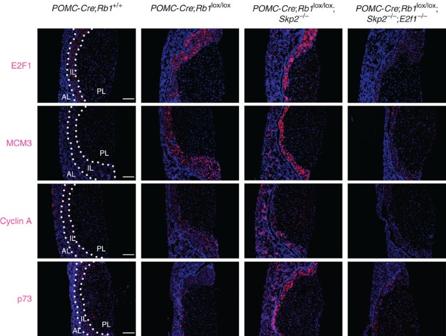Figure 3:E2f1-dependent expression of E2F target genes in pituitary IL of various genotypes. The boundary of IL is marked in pituitary sections from 2.5-week-old mice. Specific antibody IF staining was coloured in red, DAPI staining in blue. Scale bars, 50 μM. AL, anterior lobe; IL, intermediate lobe; PL, posterior lobe. Figure 3: E2f1 -dependent expression of E2F target genes in pituitary IL of various genotypes. The boundary of IL is marked in pituitary sections from 2.5-week-old mice. Specific antibody IF staining was coloured in red, DAPI staining in blue. Scale bars, 50 μM. AL, anterior lobe; IL, intermediate lobe; PL, posterior lobe. Full size image Skp2 and Rb1 co-deletion increases E2F1 on target promoters We investigated how co-deletion of Skp2 and Rb1 led to further increased expression of E2F1 target genes. pRb binds to E2Fs to bring repressive chromatin-modifying proteins to E2F target gene promoters. Phosphorylation of pRb by various cyclin/Cdks dissociates pRb from E2Fs and E2F target gene promoters. ‘Freed’ E2Fs bound on E2F target gene promoters then activate gene expression. Since Rb1 deletion is complete inactivation of pRb, other mechanisms must be involved to further increase E2F1 target gene expression by Skp2 co-deletion. Cyclin A binds the RxL domain in the amino terminus of E2F1 to inhibit E2F1’s DNA binding and transactivation activity [15] , [17] , [18] . With respect to E2F’s DNA-binding activity, E2F4 generally occupies E2F target gene promoters during G0 and G1 corresponding to repression of E2F target genes. At G1 to S phase progression, E2F4 occupancy is replaced by E2F1 coincident with expression of E2F target genes [37] , [38] . Whether E2F1 ‘freed’ from repression by pRb binds more actively to its target promoters is unknown. We determined how deletion of Rb1 affected E2F target gene promoter occupancy by E2F1. 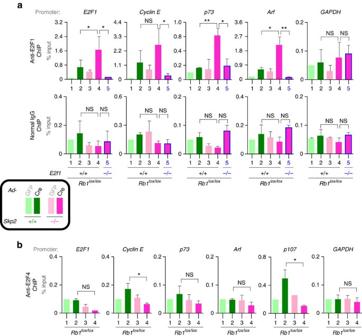Figure 4: Effects ofRb1deletion andSkp2andRb1co-deletion on promoter occupancy by E2F1 and E2F4. (a) E2F1 ChIP experiment with MEFs of the indicated genotypes. Note that lanes 5 were included to control for the anti-E2F1 antibody. (b) E2F4 ChIP experiment with MEFs of the indicated genotypes. ‘% Input’ is used to present abundance of E2F1 and E2F4 on target promoters. Data are expressed as average (mean)±s.e.m. Unpairedt-tests were performed, NS,P>0.05, *P<0.05, **P<0.01. Figure 4a shows E2F1 chromatin immunoprecipitation (ChIP) assays on promoters of E2F1, cyclin E, p73 and Arf. GAPDH promoter was included for comparison. E2f1 KO was used to control for the anti-E2F1 antibody (column 5). ‘% Input’ of anti-E2F1 ChIP on each promoters in each MEFs was compared with the ‘% input’ from WT MEFs. Normal rabbit IgG was used in a parallel set for further comparison. Columns 1 and 2 show the effect of Rb1 deletion. E2F1 occupancy on the promoters of E2F1, cyclin E, p73 and Arf all increased, with E2F1 binding to cyclin E promoter increasing the most at 10-fold. These findings suggest that ‘freed’ E2F1 could bind more actively to target promoters and more E2F1 occupancy on E2F target promoters could contribute to increased expression of E2F target genes following Rb1 deletion. We used E2F4 ChIP to provide comparison ( Fig. 4b ). Since E2F4 is preferentially bound by Rb family member p107/130 for repression, E2F4 occupancy on these promoters increased in smaller degrees by Rb1 deletion. E2F4 occupancy increased more on p107 promoters, which might explain the smaller degrees of compensatory p107 upregulation following acute Rb1 deletion [23] . Figure 4: Effects of Rb1 deletion and Skp2 and Rb1 co-deletion on promoter occupancy by E2F1 and E2F4. ( a ) E2F1 ChIP experiment with MEFs of the indicated genotypes. Note that lanes 5 were included to control for the anti-E2F1 antibody. ( b ) E2F4 ChIP experiment with MEFs of the indicated genotypes. ‘% Input’ is used to present abundance of E2F1 and E2F4 on target promoters. Data are expressed as average (mean)±s.e.m. Unpaired t -tests were performed, NS, P >0.05, * P <0.05, ** P <0.01. Full size image Figure 4a , pink columns 3 and 4 show the same ChIP experiments with Skp2 KO and Skp2;Rb1 DKO MEFs. Co-deletion of Skp2 and Rb1 induced more E2F1 occupancy to these promoters than deletion of Rb1 (green columns 1 and 2). In contrast, there was a general decrease in E2F4 occupancy on them (see the same comparisons in Fig. 4b ). Thus, more recruitment of E2F1 together with more replacement of E2F4 could explain the further increased expression from these promoters in Skp2;Rb1 DKO MEFs. Skp2 and Rb1 co-deletion decreases cyclin A on promoters Next, we investigated the mechanisms for increased E2F1 recruitment to its target promoters in Skp2;Rb1 DKO MEFs. Increased E2F1 protein levels ( Fig. 2b ) could explain its increased promoter occupancy, and increased E2F1 recruitment could explain increased E2F1 expression. To break this circular relationship, we sought to identify another property to explain the increased promoter occupancy by E2F1. We explored the relationship between cyclin A and E2F1 as described in the Introduction. In vitro , purified cyclin A/Cdk2-E2F1/DP1 complex was able to bind DNA; the kinase reaction then reduced this binding [18] . The best-established ubiquitination substrate of SCF Skp2 is p27, and p27 can compete against E2F1 for binding to cyclin A through the shared RxL motifs [39] , [40] . With co-immunoprecipitation experiments, we show that more cyclin A are bound by p27 in Skp2;Rb1 DKO MEFs than in Rb1 KO MEFs ( Fig. 5a , lanes 3 and 4), apparently owing to increased p27 in the former cells (lanes 1 and 2). p27 also bound more cyclin E and Cdk2, further suggesting that more cyclin A-p27 binding was due to more p27 in Skp2;Rb1 DKO MEFs. The paraformaldehyde crosslinking step in ChIP assays preserves protein–protein interactions before cell lysis, and real-time PCR provides quantitative measurement. ChIP assays also measure cyclin A–E2F1 interaction in the functional context of E2F1 binding to target promoters. We next attempted cyclin A ChIP to study its binding to and regulation of E2F1. We found that cyclin A was recruited to promoters of E2F1, p73 and Arf, but not GAPDH, following Rb1 deletion ( Fig. 5b , green columns 1 and 2). This cyclin A recruitment to E2F target promoters was largely (p73 promoter) or completely (E2F1 and Arf promoters) abolished by additional deletion of E2f1 (columns 5), indicating that cyclin A was recruited to these promoters via E2F1 (and possibly also E2F2 and 3, which also bind cyclin A). Normal IgG ChIP with the same samples provided a background comparison for the specific pattern of cyclin A ChIP. These results demonstrated that cyclin A-bound E2F1 can bind its target promoters and cyclin A ChIP can be used to detect cyclin A-E2F1 binding in live cells. This assay, however, did not address whether cyclin A-bound E2F1 binds to target promoters less actively. 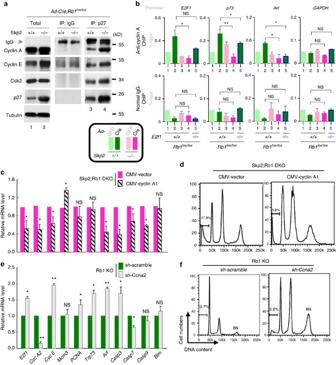Figure 5: More p27-cyclin A complex and less E2F1-cyclin A on target promoters in Skp2;Rb1 DKO MEFs than in Rb1 KO MEFs. (a) Representative (out of three) immunoprecipitation of p27 to detect p27-bound cyclin A, cyclin E and Cdk2 by western blot in Rb1 KO and Skp2;Rb1 DKO MEFs. (b) Cyclin A ChIP experiment with MEFs of the indicated genotypes quantified by qPCR and presented by % input. Note that lanes 5 were included to test whether the recruitment of cyclin A to the promoters was dependent onE2f1. (c,d) Skp2;Rb1 DKO MEFs were transduced with lentiviruses expressing cyclin A1 as indicated for 3–4 days. RT–qPCR results were normalized with GAPDH and presented as relative to the values from CMV-Vector transduced cells. Parallel cells were subject to fluorescence-activated cell sorting (FACS) analysis for sub-G1 fraction. (e,f) Rb1 KO MEFs were transduced with lentiviruses expressing short hairpin RNA targeting cyclin A2 as indicated for 3 days, and used for RT–qPCR to determine effects of cyclin A knockdown on gene expression, and FACS to determine the sizes of sub-G1 fraction in the indicated cells. Data are expressed as average (mean)±s.e.m. Unpairedt-tests were performed, NS,P>0.05, *P<0.05, **P<0.01. Figure 5: More p27-cyclin A complex and less E2F1-cyclin A on target promoters in Skp2;Rb1 DKO MEFs than in Rb1 KO MEFs. ( a ) Representative (out of three) immunoprecipitation of p27 to detect p27-bound cyclin A, cyclin E and Cdk2 by western blot in Rb1 KO and Skp2;Rb1 DKO MEFs. ( b ) Cyclin A ChIP experiment with MEFs of the indicated genotypes quantified by qPCR and presented by % input. Note that lanes 5 were included to test whether the recruitment of cyclin A to the promoters was dependent on E2f1 . ( c , d ) Skp2;Rb1 DKO MEFs were transduced with lentiviruses expressing cyclin A1 as indicated for 3–4 days. RT–qPCR results were normalized with GAPDH and presented as relative to the values from CMV-Vector transduced cells. Parallel cells were subject to fluorescence-activated cell sorting (FACS) analysis for sub-G1 fraction. ( e , f ) Rb1 KO MEFs were transduced with lentiviruses expressing short hairpin RNA targeting cyclin A2 as indicated for 3 days, and used for RT–qPCR to determine effects of cyclin A knockdown on gene expression, and FACS to determine the sizes of sub-G1 fraction in the indicated cells. Data are expressed as average (mean)±s.e.m. Unpaired t -tests were performed, NS, P >0.05, * P <0.05, ** P <0.01. Full size image On this basis, we performed the same cyclin A ChIP assay with Skp2 KO and Skp2;Rb1 DKO MEFs ( Fig. 5b , pink columns 3 and 4). The results reveal that co-recruitment of cyclin A to the same promoters did not increase in Skp2;Rb1 DKO MEFs, but showed some decrease. Significantly, this decreases in cyclin A co-recruitment to E2F target promoters occurred with further increased E2F1 recruitment to these promoters in the same cells ( Fig. 4a , pink columns 3 and 4). Furthermore, cyclin A protein was equally abundant in Rb1 KO MEFs (in which cyclin A was recruited to E2F1 target promoters) and Skp2;Rb1 DKO MEFs (in which cyclin A was not recruited; Fig. 2b ). This set of contrasting data suggested that, in Skp2;Rb1 DKO MEFs, the high amounts of p27-cyclin A complexes prevented cyclin A from binding to E2F1, and the cyclin A-unbound E2F1 bound more actively to its target promoters to increase target gene expression. We next determined the effects of increasing and lowering cyclin A levels to complement findings from ChIP experiments. We overexpressed cyclin A in Skp2;Rb1 DKO MEFs to counter the higher levels of p27 in them, and found that it repressed the expression of E2F target genes and reduced apoptosis ( Fig. 5c,d ), largely reversing the effects of Skp2 co-deletion. On the other hand, when we knocked down cyclin A in Rb1 KO MEFs, we increased the expression of E2F target genes and increased apoptosis ( Fig. 5e,f ). The accumulation of 8N cells further revealed an important role of cyclin A in mitosis in Rb1 KO MEFs. A second cyclin A knockdown hairpin reduced cyclin A expression less efficiently and showed less effects ( Supplementary Fig. 4a,b ). In comparison, knockdown of cyclin A, or cyclin E, in Skp2;Rb1 DKO MEFs did not increase E2F target gene expression or apoptosis ( Supplementary Fig. 4c,d ), probably because cyclin A in these cells was already prevented from inhibiting E2F1 by high amounts of p27. These findings suggest that Skp2 maintains cyclin A at high levels of activity to reduce expression of E2F target genes and reduce apoptosis when Rb1 is deleted. p27T187A KI reproduces effects of Skp2 KO with Rb1 deletion SCF Skp2 has a growing list of substrates in addition to p27. To determine whether p27 stabilization was the mechanism used in Skp2;Rb1 DKO MEFs to dissociate cyclin A–E2F1 interaction, we generated p27 T187A/T187A MEFs to substitute for Skp2 KO MEFs. In the following text, p27 T187A/T187A is abbreviated to AA. As shown in Fig. 6a , E2F1 binding to target promoters (E2F1, cyclin E, p73, Arf, but not GAPDH) increased in Rb1 KO MEFs (green columns) and increased further in AA;Rb1 KO MEFs (brown columns), while cyclin A co-recruitment ( Fig. 6b ) increased in Rb1 KO MEFs but increased less in AA;Rb1 KO MEFs. Parallel data from normal IgG ChIP showed background signals without specific patterns ( Supplementary Fig. 5a ). These results mimicked findings with Rb1 KO and Skp2;Rb1 DKO MEFs shown in Figs 4a and 5b . 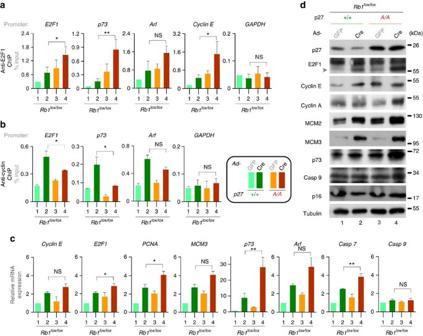Figure 6:p27T187Aknockin phenocopiesSkp2KO in Rb1 KO MEFs. (a,b) E2F1 ChIP and cyclin A ChIP experiments of the indicated MEFs. Note that brown colours replace pink colours to indicate thatp27T187A/T187AreplacesSkp2−/−. (c,d) Parallel samples were used for RT–qPCR and western blot to determine relative mRNA and protein levels, respectively, of the indicated genes. Data are expressed as average (mean)±s.e.m. Unpairedt-tests were performed, NS,P>0.05, *P<0.05, **P<0.01. Figure 6: p27T187A knockin phenocopies Skp2 KO in Rb1 KO MEFs. ( a , b ) E2F1 ChIP and cyclin A ChIP experiments of the indicated MEFs. Note that brown colours replace pink colours to indicate that p27 T187A/T187A replaces Skp2 −/− . ( c , d ) Parallel samples were used for RT–qPCR and western blot to determine relative mRNA and protein levels, respectively, of the indicated genes. Data are expressed as average (mean)±s.e.m. Unpaired t -tests were performed, NS, P >0.05, * P <0.05, ** P <0.01. Full size image The similarity between AA and Skp2 KO extended to the effects on mRNA expression. Combining Rb1 deletion with AA further increased mRNA expression of proliferative ( cyclin E , E2F1 , PCNA and MCM3 ) and apoptotic ( p73 , Arf and Casp7 ) genes ( Fig. 6c ). Of note, further increases in proliferative genes were smaller than those in apoptotic genes in AA;Rb1 KO MEFs, while they were similar in Skp2;Rb1 DKO MEFs ( Fig. 2a ). At the protein level, further increases in E2F1 in Skp2;Rb1 DKO MEFs over Rb1 KO MEFs ( Fig. 2b , lanes 2 and 4) was reproduced in AA;Rb1 KO MEFs ( Fig. 6d , lanes 2 and 4), indicating that the further increases in E2F1 protein observed in Skp2;Rb1 DKO MEFs was not due to the lack of Skp2-mediated E2F1 protein ubiquitination. With the same analysis, we could conclude that the further increases in cyclin E protein in Skp2;Rb1 DKO MEFs was in part due to lack of Skp2-mediated ubiquitination, since cyclin E protein was not further increased in AA;Rb1 KO MEFs. Also with this analysis, the further increases in p73 and cyclin A proteins in AA;Rb1 KO MEFs identified p27 stabilization as the cause. Finally, AA;Rb1 KO MEFs contained eight times more apoptotic cells than AA MEFs ( Supplementary Fig. 5b ). This line of AA MEF studies strongly suggests that it was the increase in p27 protein that led to the dissociation of cyclin A-E2F1 binding, increased binding of cyclin A-unbound E2F1 to target promoters, further increases in their expression at mRNA and protein levels and increased apoptosis. Convert E2F1 from proliferative to apoptotic effector Following the biochemical studies above, we determined the role of E2f1 in Rb1 and Skp2 co-deletion-induced apoptosis. We found that infection of Skp2 −/− ;Rb1 lox/lox ;E2f1 −/− MEFs by Ad-Cre induced apoptosis in 3.0% of the cells, compared with 1.1% apoptosis by Ad-GFP in parallel infections ( Supplementary Fig. 6 ). Compared with 19% apoptosis when Rb1 was deleted in Skp2 −/− ;Rb1 lox/lox MEFs ( Fig. 1a ), this finding suggested that E2F1 is a major apoptosis inducer following co-deletion of Rb1 and Skp2 . In Rb1 -deficient pituitary IL tumorigenesis, the role of deregulated E2F1 was proliferative, as combined deletion of E2f1 reduced IL mass [3] . Our findings above suggested that the absence of the deregulated Skp2 might convert the deregulated E2F1 from proliferative to apoptotic following Rb1 loss. We next compared the effects of E2f1 deletion on pituitary IL in POMC-Cre;Rb1 lox/lox and Skp2 −/− ;POMC-Cre;Rb1 lox/lox mice. We measured Ki67 and TUNEL staining in pituitaries at the age of 2.5 weeks. Co-deletion of Skp2 did not reduce Ki67 staining but increased TUNEL staining; additional deletion of E2f1 significantly reduced Ki67 and TUNEL staining ( Supplementary Fig. 7a ). Thus, E2F1 was required for both proliferation and apoptosis in the Skp2 −/− ;POMC-Cre;Rb1 lox/lox IL. At the age of 7 weeks, POMC-Cre;Rb1 lox/lox mice showed nodular transformation across the entire IL, whereas the IL in Skp2 −/− ;POMC-Cre;Rb1 lox/lox mice had been ablated to a layer of one-cell thick ( Fig. 7a–c ). Deletion of E2f1 significantly reduced the mass of the tumorigenic IL such that the IL of 7-week-old POMC-Cre;Rb1 lox/lox ;E2f1 −/− mice appeared similar to that in WT mice ( Fig. 7d ). In contrast, deletion of E2f1 significantly increased the mass of the ablated IL to that of a WT IL in Skp2 −/− ;POMC-Cre;Rb1 lox/lox ;E2f1 −/− mice ( Fig. 7e ), demonstrating, instead, an apoptotic role of E2F1. 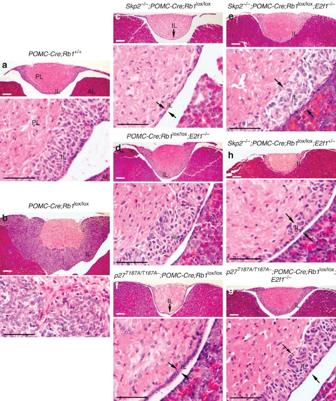Figure 7:Skp2KO orp27T187Aknockin converts E2F1’s role inRb1-deficient pituitary IL from proliferative to apoptotic. Presented are haematoxylin and eosin stains of the pituitary coronal sections. For each pituitary, a low magnification view (upper) shows the entire pituitary IL and a high magnification one (lower) shows a segment of the IL in more detail. Animals were about 7 weeks old. Scale bars, 100 μM. AL, anterior lobe; IL, intermediate lobe; PL, posterior lobe. Figure 7: Skp2 KO or p27T187A knockin converts E2F1’s role in Rb1 -deficient pituitary IL from proliferative to apoptotic. Presented are haematoxylin and eosin stains of the pituitary coronal sections. For each pituitary, a low magnification view (upper) shows the entire pituitary IL and a high magnification one (lower) shows a segment of the IL in more detail. Animals were about 7 weeks old. Scale bars, 100 μM. AL, anterior lobe; IL, intermediate lobe; PL, posterior lobe. Full size image We extended this line of pituitary studies to Skp2 target p27. As shown in Supplementary Fig. 7b , at 2.5 weeks of age, combining Rb1 deletion with p27 T187A/T187A knockin further increased expression of MCM3, cyclin A and p73, which were then reduced by additional deletion of E2f1 . Ki67 and TUNEL showed the same pattern of changes (compare Supplementary Fig. 7c with 7a). When p27 T187A/T187A ;POMC-Cre;Rb1 lox/lox mice aged to 7 weeks, the pituitary IL was also nearly ablated ( Fig. 7f ), but reverted to WT sizes in p27 T187A/T187A ;POMC-Cre;Rb1 lox/lox ;E2f1 −/− mice ( Fig. 7g ). Thus, p27 stabilization was sufficient to bring out the apoptotic activity of E2f1 . The requirement for p27 binding to cyclin A was previously addressed by mutating p27’s RxL motif to AxA. p27AxA developed larger body sizes and pituitary tumours like p27 KO, confirming that binding to cyclin/Cdk is the major function of p27 (ref. 41 ). Further, abolishing p27’s ability to bind cyclin/Cdk impaired its phosphorylation by cyclin/Cdk and increased its protein levels, suggesting that without p27-cyclin/Cdk-binding, pituitary tumorigenesis can occur even when p27 protein levels were increased [41] . We recently showed that deletion of p27 in Skp2 −/− ;POMC-Cre;Rb1 lox/lox ;p27 −/− mice completely abolished apoptosis and induced robust pituitary tumorigenesis [36] , suggesting that p27 function is necessary downstream of Skp2 deletion to induce apoptosis and block Rb1 -deficient pituitary tumorigenesis. We also assessed whether the apoptotic role of E2F1 in Skp2 −/− ;POMC-Cre;Rb1 lox/lox pituitary was dependent on its dosage. Reduction of E2f1 gene dosage to half still ameliorated the ablation of the IL by Skp2 KO ( Fig. 7h ), although not to the level by E2f1 KO. Thus, the apoptotic activity of the further activated E2F1 is critically dependent on its levels. KO of Skp2 or E2f1 , or knockin of p27 T187A showed no effects on the pituitary IL ( Supplementary Fig. 8 ). Skp2-cyclin A binding enhances Rb1 -deficient tumorigenesis The above studies identified an Skp2-p27-cyclin A-E2F1 pathway that prevents apoptosis in Rb1 -deficient tumorigenesis. Intriguingly, Skp2 also directly binds cyclin A in cancer cells (as described in the Introduction). We previously determined that Skp2 binding to cyclin A competes against p27 binding to cyclin A but not against E2F1 binding to cyclin A since Skp2 does not use an RxL motif to bind cyclin A [42] . Thus, Skp2-cyclin A binding might also promote cyclin A-E2F1 binding (since cyclin A is protected from binding to p27) and therefore restrain E2F1 activity following Rb1 loss. Lack of Skp2-cyclin A binding might act in synergy with and/or independent of increase in p27 to further activate E2F1 in Skp2;Rb1 DKO cells to induce apoptosis. To gain a more complete understanding of Skp2 functions, we determined the significance of Skp2-cyclin A binding by abolishing Skp2’s ability to bind cyclin A. We previously mapped the cyclin A-binding sequences on Skp2 to between residues 40 and 60, and generated a Skp2 mutant that cannot bind cyclin A by mutating the four conserved residues [42] (the Skp2AAAA mutant, Fig. 8a ). We showed that Skp2AAAA did not affect Skp2’s ability to complex with Skp1-Cul1-Roc1, and the resulting SCF Skp2AAAA complex was fully active in mediating p27 polyubiquitination. Skp2AAAA also localized to the nucleus and can be phosphorylated by cyclin A/Cdk2 like WT Skp2 (ref. 42 ). APC Cdh1 ubiquitin ligase can promote Skp2 degradation [43] , [44] ; Skp2AAAA was found to bind less Cdh1 (ref. 45 ). 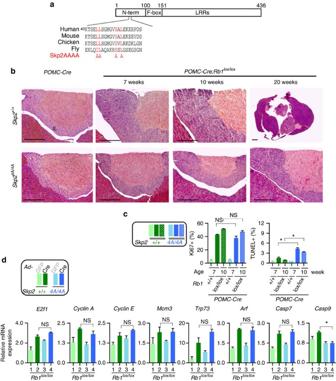Figure 8:Skp2AAAAknockin delaysRb1-deficient pituitary tumorigenesis by increasing apoptosis. (a) Cartoon illustration of the Skp2AAAA mutant. (b) Haematoxylin and eosin-stained pituitary sections of the indicated genotypes at the indicated ages. At 20 weeks, all fivePOMC-Cre;Rb1lox/loxmice, but only one in fiveSkp24A/4A;POMC-Cre;Rb1lox/loxmice had gross pituitary tumours. The other four showed thickened IL. (c) Quantification of Ki67 staining and TUNEL staining in IL of the indicated genotypes. (d) RT–qPCR of E2F target gene expression in indicated MEFs. Note that blue colours replace pink colours to indicate thatSkp4A/4AreplacesSkp2−/−. Data are expressed as average (mean)±s.e.m. Unpairedt-tests were performed, NS,P>0.05, *P<0.05. Scale bars, 200 μM. IL, intermediate lobe. Figure 8: Skp2AAAA knockin delays Rb1 -deficient pituitary tumorigenesis by increasing apoptosis. ( a ) Cartoon illustration of the Skp2AAAA mutant. ( b ) Haematoxylin and eosin-stained pituitary sections of the indicated genotypes at the indicated ages. At 20 weeks, all five POMC-Cre;Rb1 lox/lox mice, but only one in five Skp2 4A/4A ;POMC-Cre;Rb1 lox/lox mice had gross pituitary tumours. The other four showed thickened IL. ( c ) Quantification of Ki67 staining and TUNEL staining in IL of the indicated genotypes. ( d ) RT–qPCR of E2F target gene expression in indicated MEFs. Note that blue colours replace pink colours to indicate that Skp 4A/4A replaces Skp2 −/− . Data are expressed as average (mean)±s.e.m. Unpaired t -tests were performed, NS, P >0.05, * P <0.05. Scale bars, 200 μM. IL, intermediate lobe. Full size image We generated a knockin mouse in which the Skp2AAAA mutations were introduced into the mouse Skp2 gene, creating Skp2 4A ( Supplementary Fig. 9 ). Mating Skp2 4A/+ mice produced Skp2 4A/4A mice with Mendelian ratios and these mice appeared normal. Skp2AAAA expressed in Skp2 4A/4A MEFs migrated slightly larger and at slightly lower levels than Skp2 in WT MEFs, while cyclin A and p27 protein levels were not different from those in WT MEFs ( Supplementary Fig. 9c ). We generated Skp2 4A/4A ;POMC-Cre;Rb1 lox/lox mice and found that Rb1 -deficient pituitary tumorigenesis in them was slower than in POMC-Cre;Rb1 lox/lox mice ( Fig. 8b ). By 20 weeks, all five POMC-Cre;Rb1 lox/lox mice, but only one in five Skp2 4A/4A ;POMC-Cre;Rb1 lox/lox mice had gross pituitary tumours. The other four showed only thickened IL ( Fig. 8b ). Skp2AAAA knockin, like Skp2 KO or p27T187A knockin, did not reduce proliferation in pituitary IL, but increased apoptosis in it ( Fig. 8c , blue columns). However, the extent of IL apoptosis was smaller in Skp2 4A/4A ;POMC-Cre;Rb1 lox/lox pituitary than in Skp2 −/− ;POMC-Cre;Rb1 lox/lox or p27 T187A/T187A ;POMC-Cre;Rb1 lox/lox pituitaries ( Supplementary Fig. 7a,c ). In MEFs, combining Skp2AAAA knockin in 4A4A;Rb1 KO MEFs did not in general induce further increased expression of a similar set of E2F target genes, except for p73, which nonetheless did not reach statistical significance ( Fig. 8d ). These findings reveal that the cyclin A-binding activity of Skp2 is important in providing survival support for Rb1 -deficient pituitary tumorigenesis, but reaffirm that the major functional mechanism of Skp2 in promoting survival following Rb1 deletion is to mediate p27 degradation by the SCF Skp2 ubiquitin ligase. Studies to understand how pRb suppresses tumorigenesis have identified a growing list of more than 200 pRb targets [46] , [47] . Many of them demonstrated physiologically relevant roles in Rb1 -deficient tumorigenesis since targeted deletion of the encoding gene delayed pituitary tumorigenesis in Rb1 +/− mice [3] , [4] , [5] , [48] , [49] , [50] , [51] . The pRb target Skp2 is an exception. Deletion of Skp2 prevented pituitary tumorigenesis in Rb1 +/− mice, and reduced the entire IL to a layer of one-cell thick in POMC-Cre;Rb1 lox/lox mice, revealing a surprisingly effective anti- Rb1 -deficient tumorigenesis mechanism [13] . We now shed light on how this mechanism operates. The most accepted model for how Rb1 deletion induces tumorigenesis is that loss of pRb activates E2F target gene expression. Our finding that combined deletion of Skp2 further increased the expression of the activated E2F target genes provided a first key insight. Oncogenic events often induce anti-oncogenic responses that safeguard against tumorigenesis [52] . The finding that activated E2F1 can induce apoptosis predicted, but was unable to subsequently demonstrate, a pRb-E2F1-apoptosis safeguard against Rb1 -deficient tumorigenesis. By further activating E2F target gene expression, combined Skp2 deletion might have unmasked this safeguard. We show that E2F1 and cyclin A together binds more E2F target gene promoters following Rb1 deletion. With Skp2 and Rb1 co-deletion, p27 binds more cyclin A; cyclin A is no longer co-recruited with E2F1 to target gene promoters, while E2F1 binds further more to these promoters. Importantly, these effects of Skp2 KO were phenocopied by p27T187A knockin. In the absence of Skp2 or presence of p27T187A, combining E2f1 deletion with Rb1 deletion increased IL mass. These data demonstrate that increases in p27 following Skp2 deletion negated cyclin A’s ability to limit E2F1 activity, and the unrestrained E2F1 activates the pRb-E2F1-apoptosis safeguard (cartoon summary in Fig. 9 ). Next, it is important to determine whether cyclin A limits E2F1 activity by phosphorylating it (after binding to it), what residues of E2F1 and its partner DP1 are phosphorylated and what is the physiological significance of their phosphorylation compared with physical binding alone. It is also important to determine the targets of E2F1 affecting this safeguard. In our preliminary studies, knockdown of p73 in Skp2;Rb1 DKO MEFs significantly reduced apoptosis, suggesting an effective E2F1-p73 pathway for this safeguard for in vivo validation. 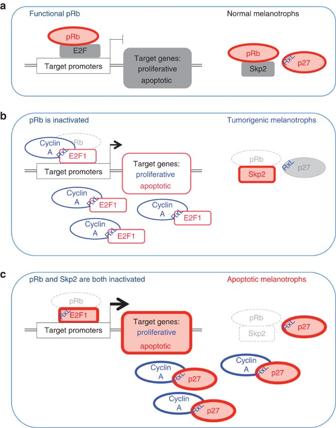Figure 9: Graphic summary for how deregulation of Skp2 limits E2F1 activity to promote tumorigenesis followingRb1deletion. (a) Normally, pRb binds and represses E2F transcription factors to repress expression of E2F target genes. pRb also binds and represses Skp2 to inhibit p27 degradation. (b) Following loss of pRb, E2F1 becomes active, or de-repressed, to transactivate, or de-repress, target gene expression; moreover, Skp2 is activated to reduce p27 protein amount. In this situation, E2F1 activity is restrained since E2F1 is bound to and repressed by cyclin A, leading to tumorigenesis. (c) WhenSkp2is co-deleted withRb1, p27 protein amounts increase, and p27 competes with E2F1 for binding to cyclin A. When E2F1 is not bound by cyclin A, it binds target promoters and activates target genes more potently, leading to apoptotic ablation of melanotrophs. Molecules and actions are active when written in bold red and coloured with red with thick red border. Inactive and repressed states are grey and written in regular black. Restrained E2F1 and target gene expression are written in regular red, coloured in white with regular red borders. Cyclin A is one of the proliferative genes in blue. Figure 9: Graphic summary for how deregulation of Skp2 limits E2F1 activity to promote tumorigenesis following Rb1 deletion. ( a ) Normally, pRb binds and represses E2F transcription factors to repress expression of E2F target genes. pRb also binds and represses Skp2 to inhibit p27 degradation. ( b ) Following loss of pRb, E2F1 becomes active, or de-repressed, to transactivate, or de-repress, target gene expression; moreover, Skp2 is activated to reduce p27 protein amount. In this situation, E2F1 activity is restrained since E2F1 is bound to and repressed by cyclin A, leading to tumorigenesis. ( c ) When Skp2 is co-deleted with Rb1 , p27 protein amounts increase, and p27 competes with E2F1 for binding to cyclin A. When E2F1 is not bound by cyclin A, it binds target promoters and activates target genes more potently, leading to apoptotic ablation of melanotrophs. Molecules and actions are active when written in bold red and coloured with red with thick red border. Inactive and repressed states are grey and written in regular black. Restrained E2F1 and target gene expression are written in regular red, coloured in white with regular red borders. Cyclin A is one of the proliferative genes in blue. Full size image There are a number of other mechanisms for negative regulation of E2F1. Skp2 binds and protects cyclin A from p27 binding while still allowing E2F1 binding [42] . By generating a Skp2AAAA knockin mouse, we demonstrate that Skp2–cyclin A interaction also provides survival support in Rb1 -deficient pituitary tumorigenesis, but to a lesser degree than Skp2 KO or p27T187A knockin. Serum starvation or inhibition of PI3K-Akt signalling is required for the apoptotic activity of overexpressed E2F1, because PI3K-Akt signalling represses a group of E2F1 target genes [53] , [54] . Skp2 can activate Akt in response to EGF signalling [55] . Our preliminary studies show that Skp2 KO and Skp2;Rb1 DKO MEFs responded normally to serum starvation restimulation with Akt phosphorylation. Of the four validated genes repressed by serum-PI3K [53] , AMPKα2 and Cyp26b1 responded with increases in Rb1 KO MEFs (relative to WT MEFs) and further increases in Skp2;Rb1 DKO MEFs (relative to Rb1 KO MEFs), while Nr4a2 and p27 showed no changes. SCF Skp2 (ref. 19 ), SCF Slmb [20] and CRL4 Cdt2 (ref. 21 ) can mediate degradation of E2F1. In our studies, protein levels of E2F1 were correlated with its mRNA levels. Nevertheless, when combined, the above mechanisms could more significantly contribute to Rb1 -deficient tumorigenesis. Impressively, the ability of the activated E2F1 to induce apoptosis is more than sufficient to block tumorigenesis since it reduced the normal structure of IL to only one-cell thick. One could imagine, then, that the ability of Rb1 deletion to induce fully penetrant pituitary tumorigenesis is an exception rather than a default. Indeed, in POMC-Cre;Rb1 lox/lox mice, Rb1 deletion in pituitary melanotrophs is tumorigenic, in hypothalamus POMC neurons is apoptotic, in POMC neurons in nucleus tractus solitaries and in postnatally born neurons in dentate gyrus are without apparent effects [56] . Furthermore, the apoptosis in POMC neurons was also due to E2F1 (ref. 56 ). It would be interesting to determine whether deletion of Rb1 can induce tumorigenesis only when Skp2 can be deregulated at the same time. Finally, the ability of E2F1 to induce apoptosis by p53-dependent and p53-independent mechanisms may extend its safeguard role to pRb and p53 doubly deficient tumours. Skp2 can inhibit acetylation and activation of p53 (ref. 57 ); however, Skp2 deletion still blocked pRb and p53 doubly deficient pituitary and prostate tumorigenesis [36] . It is likely that E2F1 might be further activated, through mechanisms described in this study, to induce apoptosis p53 independently to limit the accumulation of pRb and p53 doubly deficient neoplastic cells. Mice Rb1 lox/lox mice [23] , Pomc-Cre mice [58] , Skp2 −/− mice [22] , p27 T187A/T187A mice [59] and E2f1 −/− mice [60] have been described previously. Mice used in this study were on mixed C57BL/6J × 129Sv strain background and of both sexes. Generation of Skp2 −4A/4A mice is described below. All procedures were reviewed and approved by Einstein Animal Care Committee, conforming to accepted standards of humane animal care. The Skp2AAAA knockin cassette was constructed from the left and right arms. For the left arm, we subcloned from a Skp2 Bac plasmid pSkp2-8 XH-N, a 1.5-kb fragment, using sites Xho I and Eag I into pBluescript SKII+. We used Stratagene Site Directed Mutagenesis Kit to introduce the AAAA mutations. The resulting plasmid contained a region flanked by Eag I and Bsp EI sites, which we used to create the pBSK 1.5 kb-4A plasmid and sequence confirmed the insertion of the Skp24A mutations. We replaced the Pst I site between exons 1 and 2 with a Pst I- Not I- Sal I- Pst I DNA linker into which the ~2.5 kb neomycin resistance (NEO) cassette was inserted. For the right arm, we first replaced the Sac I site on the pBluescript SKII+ with a Sac I- Bst BI- Sac I DNA linker (this modified pBSK is called pBSK- Bst BI). We then excised the 6.1-kb right arm from Eag I to Bst BI from plasmid pSkp2-8 XH-C and cloned it into pBSK- Bst BI, resulting in pBSK 6.1. Next, we subcloned the 1.5-kb left arm without the Skp2AAAA mutations using the Xho I and Sal I into the pBSK 6.1 plasmid to create the pBSK-Skp2- Eag I- Sal I 6.1 plasmid. We then replaced the 243-bp region flanked by Sal I and Eag I with the corresponding fragment containing the Skp2AAAA mutations. We subcloned in the NEO cassette using the created Not I and Sal I sites to generate the pBSK-Skp2-1.5-4A-6.1-243 NEO plasmid. pBSK-Skp2-1.5-4A-6.1-243 NEO plasmid was linearized with Kpn I and electroporated into WW6 embryonic stem cells by the Einstein Transgenic Mouse Core. G418 resistant cells were selected in 250 μg ml −1 G418, leading to a total of ~400 embryonic stem cell colonies successfully picked and frozen. We isolated genomic DNA from a portion of each colony, screened each clone by PCR (using primers, bf Xho I-5 and ins cas-3, outside the homologous recombination region and within the NEO cassette, yielding an ~1.3 kb product). Three positive colonies were identified: clone 16,119 and 175. Clone 16 was confirmed by Southern blot analysis using a genomic DNA probe outside the targeting vector to detect the expected 9.6-kb homologously recombined fragment. We used clone 16 to generate chimeric mice. Male mouse showing germline transmission was mated with ZP-3-Cre female mice to remove the neomycin cassette. Female progeny were checked using PCR analysis to verify whether the neomycin cassette has been excised. The PCR primers used are 355 Pst I and Aft Eag I that flank the neomycin cassette and contain the four Skp24A mutations. The resulting PCR products yielded the expected sizes of 392 bp (contains a 30-bp residual loxP site after Cre-mediated excision plus mutations) and 362 bp (a WT product without a loxP site) bands. The 392-bp product was sequenced and yielded the lone loxP site as well as the four-alanine mutations within exon 2. The resulting mice, Skp2 4A/+ were mated for five generations with C57/Bl6 mice. MEFs MEFs were isolated from E13.5 embryos and cultured in 10% fetal bovine serum DMEM [61] . Genotyping used primers listed in Supplementary Table 1 . Deletion of Rb1 in Rb1 lox/lox MEFs was achieved with infection by adenoviruses expressing GFP or Cre at a multiplicity of infection of 30–120 particle units for 8 h at 37 °C. Lentivirus vectors expressing sh- Ccna2 (TRCN0000077764, TRCN0000077765), sh- Ccne1 (TRCN0000077774, TRCN0000077776) and CMV- CCNA1 (open reading frame clone accession: DQ894488) were purchased from Open Biosystem. Generation of lentiviral stocks and transduction of MEFs were as described [62] . RT–qPCR and western blots Cells were harvested at 16 h post plating. Total RNA was isolated with RNeasy kit (Qiagen) and reversed transcribed to complementary DNA with Superscript First Strand Synthesis System (Invitrogen). About 2.5 μg complementary DNA of each sample was used as template for real-time PCR reactions using SYBR Green dye (Applied Biosystems). Samples were run in triplicate and results were normalized with GAPDH in the same samples. The primers for RT–qPCR are listed in Supplementary Table 1 . Cell lysates were made with RIPA buffer. Fifty micrograms of total protein extract was loaded on 10% SDS gel, blotted and probed with specific antibodies. Caspase 9 (Santa Cruz Biotechnology, H170), p73 (Abcam, EP436Y) and E2F1 (Santa Cruz, c20) were used with 1:100 dilution; cyclin A (Santa Cruz, c19) and cyclin E (Santa Cruz, M20) were used with 1:200 dilution; MCM2 (BD, 610700), MCM3 (Santa Cruz Biotechnology, N19) and P53 (Cell Signalling, 1C12) were used with 1:300 dilution; PCNA (BD, 610664) and p27 (BD, 610242) were used at 1:1,500 dilution. Relative abundance of protein extract was visualized with antibody to tubulin (Sigma-Aldrich). Chromatin immunoprecipitation ChIP was performed as described [37] . In brief, about 3 × 10 6 MEFs were harvested at about passage 6 and fixed with 1% formaldehyde. After cell lysis, nuclei were separated and sonicated on ice to fragment DNA to an average length of 700 bp. Then the crossliked and sonicated chromatin was subjected to immunoprecipitation with ChIP grade antibodies: cyclin A (H-432X), E2F1 (C-20X), E2F4 (A-20X) and normal rabbit IgG (SC-2027; all from Santa Cruz Biotechnology). Following purification, about 5% of total precipitated DNA and 0.1% input were analysed by qPCR. Data were analysed as % of input. ChIP primer sequences have been listed in Supplementary Table 1 . Immunohistochemistry and immunofluorescence staining Mice were anaesthetized and perfused through the left ventricle with PBS. Stain was performed as described [13] . In brief, pituitaries were dissected out and post fixed in 4% paraformaldehyde followed by cryoprotection with 30% sucrose for 48 h. Pituitary sections of 10 μm were prepared with the use of Cryostate (Thermo Scientific). Sections were first treated with 3% H 2 O 2 to quench endogenous peroxidase, washed several times, blocked with 10% normal rabbit serum and then incubated in primary antibodies at room temperature for 1 h or at 4 °C overnight. Antibodies to E2F1 (c20), cyclin A (c19), cyclin E (M20) and Mcm3 (N19) were from Santa Cruz Biotechnology, to p73 (EP436Y) from Abcam, to Ki67 (SP6) from Thermo scientific and to cleaved caspase-3 (D175) from Cell Signaling. After wash, sections were incubated with horseradish peroxidase-conjugated secondary antibody (Perkin Elmer, NEF812001EA) at room temperature for 1 h, followed by tyramide signal amplification (Perkin Elmer NEL744). TUNEL staining was performed with Apoptosis Detection Kit (Chemicon S7101) according to the user’s manual. How to cite this article: Lu, Z. et al. Skp2 suppresses apoptosis in Rb1-deficient tumours by limiting E2F1 activity. Nat. Commun. 5:3463 doi: 10.1038/ncomms4463 (2014).